Parallel evolution of Nicaraguan crater lake cichlid fishes via non-parallel routes Fundamental to understanding how biodiversity arises and adapts is whether evolution is predictable in the face of stochastic genetic and demographic factors. Here we show rapid parallel evolution across two closely related but geographically isolated radiations of Nicaraguan crater lake cichlid fishes. We find significant morphological, ecological and genetic differentiation between ecomorphs in sympatry, reflected primarily in elongated versus high-bodied shape, differential ecological niche use and genetic differentiation. These eco-morphological divergences are significantly parallel across radiations. Based on 442,644 genome-wide single nucleotide polymorphisms, we identify strong support for the monophyly of, and subsequent sympatric divergence within, each radiation. However, the order of speciation differs across radiations; in one lake the limnetic ecomorph diverged first while in the other a benthic ecomorph. Overall our results demonstrate that complex parallel phenotypes can evolve very rapidly and repeatedly in similar environments, probably due to natural selection, yet this evolution can proceed along different evolutionary genetic routes. Twenty-five years ago Stephen Jay Gould famously proposed a thought experiment in which he argued that, were one to ‘rewind the tape of life’, evolution would not repeat itself [1] . Gould’s rationale was the importance of stochasticity and accidental events in generating biodiversity [1] . Gould’s prediction remains highly contended [2] , in part because repeated ‘natural experiments’ that might inform this debate are exceedingly rare. While Gould’s hypothesis referred to deep geological time, it is expected that, since microevolutionary processes explain macroevolutionary patterns [3] , ‘natural experiments’ at smaller geographic and shorter temporal scales should conform to Gould’s famous prediction. Because replication seems to emphasize predictability over randomness during evolution, the repeated evolution of equivalent phenotypes has long fascinated biologists. Specifically in parallel phenotypic evolution, similar morphologies evolve independently from a recent common ancestor in separate but often similar environments [4] . This is considered to be strong evidence for adaptation through Darwinian natural selection rather than by stochastic divergence and suggests somewhat deterministic evolutionary trajectories. The most famous vertebrate adaptive radiations (for example, sticklebacks, Arctic charr and whitefishes in postglacial freshwaters, anole lizards on Caribbean islands and Darwin’s finches in the Galapagos islands) are examples of parallel phenotypic evolution [4] , [5] , [6] . With the aim of understanding the extent to which there is convergence in the proximate mechanisms underlying similar adaptive outcomes, evolutionary biologists have revisited this issue with new theory and empirical methods to study repeated parallel evolution in adaptive radiations (for example, see refs 5 , 6 , 7 ). The emerging pattern suggests that divergence into parallel phenotypes may occasionally be associated with non-parallel genetic processes (for example, see refs 7 , 8 , 9 , 10 , 11 , 12 and reviewed in refs 13 , 14 ), although studies on populations in nature can rarely exclude an influence of gene flow. However, it has remained an open question as to how often parallel ecological or morphological phenotypic evolution is underlain by parallel evolutionary or genetic processes (reviewed in ref. 14 ), because settings in nature for testing the repeatability of evolution in spatially independent environments are extremely rare [4] , [5] , [15] . The young and completely isolated crater lakes along the Central America Volcanic Arc in Nicaragua (reviewed in ref. 16 ) provide an ideal ‘natural experiment’ for testing these aspects of evolutionary repeatability. Several crater lakes house populations of Midas cichlid fishes ( Amphilophus citrinellus species complex) that are recently and independently derived from generalist populations in nearby Great Lakes Managua and Nicaragua [17] ( Fig. 1a ). In only two crater lakes, Apoyo and Xiloá, small adaptive radiations of four to six described species of Midas cichlid fishes formed in <10,000 years (refs 16 , 18 , 19 ). Recent analyses suggested these two radiations show similar levels of morphological divergence from any other Midas cichlid population [16] . In addition to a flock of benthic species (‘Benthics’), each radiation harbours a single arrow-shaped or elongate limnetic species ( A. zaliosus in Apoyo [20] , [21] , A. sagittae [22] in Xiloá), a phenotype otherwise absent from other Neotropical lakes [20] . The deep, clear water of the crater lakes ( Fig. 1b,c ) may allow for new niches compared with the shallow, murky water of the ancestral Great Lakes (reviewed in ref. 16 ). 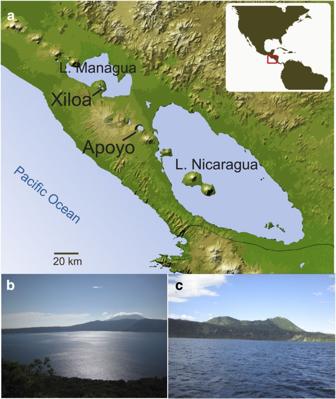Figure 1: Study area. (a) Topographic map of Nicaragua showing the location of the two crater lakes that are the focus of the present study, Xiloá and Apoyo. (b) Photograph of Apoyo and (c) Xiloá, showing the crater walls and lake landscape. Lake Apoyo was formed maximally 23 kya, >200 m deep at its maximum, with very clear water (~3.0 m secchi visibility). Lake Xiloa is 88.5 m deep at its maximum, clear watered (~2.5 m secchi visibility) and was formed maximally 6.1 kya (reviewed in ref.16). Figure 1: Study area. ( a ) Topographic map of Nicaragua showing the location of the two crater lakes that are the focus of the present study, Xiloá and Apoyo. ( b ) Photograph of Apoyo and ( c ) Xiloá, showing the crater walls and lake landscape. Lake Apoyo was formed maximally 23 kya, >200 m deep at its maximum, with very clear water (~3.0 m secchi visibility). Lake Xiloa is 88.5 m deep at its maximum, clear watered (~2.5 m secchi visibility) and was formed maximally 6.1 kya (reviewed in ref. 16 ). Full size image Here we conducted a combined assessment of morphological, ecological, population genetic and phylogenetic patterns to test whether the Midas cichlid radiations in these two crater lakes represent parallel evolution along the littoral shore to open water (benthic–limnetic) axis characteristic of freshwater fishes [4] . Criteria for parallel phenotypic evolution [14] required: (1) phenotypic and genetic divergence between ecomorphs (Benthic versus Limnetic) in sympatry, (2) equivalent ecomorphs that were (3) replicated independently across environments [4] , [23] . We find strong support for morphological, ecological and genetic divergence between Benthics and Limnetics in sympatry and evidence for parallel phenotypic evolution across the replicate crater lake radiations. However, the evolutionary genetic pattern of speciation differs between the radiations in each crater lake. Eco-morphological differentiation We found that the main body shape variation within lakes was between ecomorphs, as evidenced by a principal components analysis that separated the single Limnetic species from all Benthics along the first axis ( Fig. 2a ; Supplementary Fig. 2a ; species-level analysis in Supplementary Fig. 1 ) ( N =894). All species other than the Limnetics ( A. zaliosus in Apoyo, A. sagittae in Xiloá) overlapped or slightly separated along the second axis of variation ( Supplementary Fig. 1 ; in agreement with previous work on components of these radiations [16] , [21] , [22] ) and are combined as ‘Benthics’ for all further ecomorph-level analyses. 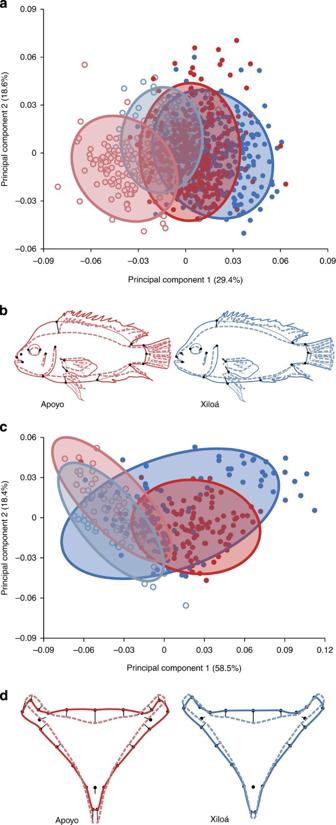Figure 2: Parallelism in eco-morphological variation of Midas cichlids across two crater lakes. (a) Body shape variation among individuals along PC1 and PC2 in both lakes withouta priorigrouping, where each dot represents an individual’s morphology as described by 18 homologous landmarks and ecomorphs are delimited by 90% probability ellipses (N=894). PC1 separates Limnetics (open circles: pink in Apoyo, light blue in Xiloá) and Benthics (closed circles: red in Apoyo, dark blue in Xiloá). (b) Comparison of shape difference between mean Benthics (dark line) and Limnetics (pale dashed line) based on discriminant function analysis (scale factor 2 for visualization). Black dots represent landmark location in Benthics and line termini the homologous location in Limnetics. Limnetics have a more elongated body form while Benthics are more high bodied and have larger heads. (c) LPJ shape variation among individuals along PC1 and PC2 in both lakes withouta priorigrouping, where each dot represents an individual’s LPJ morphological space as described by 24 landmarks and ecomorphs are delimited by 90% probability ellipses (N=297). PC1 separates Limnetics (open circle: pink in Apoyo, light blue in Xiloá) and Benthics (closed circle: red in Apoyo, dark blue in Xiloá). (d) Comparison of shape difference between mean Benthics (dark line) and Limnetics (pale dashed line) based on discriminant function analysis (scale factor 2 for visualization). Black dots represent mean landmark location in Benthics and line termini the homologous mean location in Limnetics. Note that forbandd, the lines connecting the landmarks are only indicative of inter-landmark shape. Figure 2: Parallelism in eco-morphological variation of Midas cichlids across two crater lakes. ( a ) Body shape variation among individuals along PC1 and PC2 in both lakes without a priori grouping, where each dot represents an individual’s morphology as described by 18 homologous landmarks and ecomorphs are delimited by 90% probability ellipses ( N =894). PC1 separates Limnetics (open circles: pink in Apoyo, light blue in Xiloá) and Benthics (closed circles: red in Apoyo, dark blue in Xiloá). ( b ) Comparison of shape difference between mean Benthics (dark line) and Limnetics (pale dashed line) based on discriminant function analysis (scale factor 2 for visualization). Black dots represent landmark location in Benthics and line termini the homologous location in Limnetics. Limnetics have a more elongated body form while Benthics are more high bodied and have larger heads. ( c ) LPJ shape variation among individuals along PC1 and PC2 in both lakes without a priori grouping, where each dot represents an individual’s LPJ morphological space as described by 24 landmarks and ecomorphs are delimited by 90% probability ellipses ( N =297). PC1 separates Limnetics (open circle: pink in Apoyo, light blue in Xiloá) and Benthics (closed circle: red in Apoyo, dark blue in Xiloá). ( d ) Comparison of shape difference between mean Benthics (dark line) and Limnetics (pale dashed line) based on discriminant function analysis (scale factor 2 for visualization). Black dots represent mean landmark location in Benthics and line termini the homologous mean location in Limnetics. Note that for b and d , the lines connecting the landmarks are only indicative of inter-landmark shape. Full size image Body shape differed between ecomorphs ( P <0.0001, permutation test for Procrustes distances among groups, N =894; Supplementary Table 1 ), primarily because of body height compression and an elongated caudal peduncle in the Limnetics ( Fig. 2b ) (that is, higher elongation index; Supplementary Fig. 3a ). These elongate versus high-bodied physiques are generally associated with different swimming performances and closely linked to ecological niche across freshwater fishes [24] . The ecological niche of cichlid fishes is also reflected in characteristic morphologies of their trophic apparatus, chiefly the lower pharyngeal jaw (LPJ) [25] , which enables effective processing of prey items [26] . LPJ shape differed between Benthics and Limnetics in both lakes ( P <0.0001, permutation test for Procrustes distances among groups, N =297) ( Fig. 2c ; Supplementary Fig. 2b ; Supplementary Table 1 ). Benthics’ LPJs were more robust, with thicker horns and a larger dentigerous area ( Fig. 2d ). Benthics and Limnetics also differed in LPJ size and weight, with Benthic LPJs being wider, longer, deeper and heavier in both radiations ( Supplementary Fig. 3d–g ). Ecological differentiation Ecological divergence within lakes was quantified directly from stable isotopes that vary depending on an individual’s foraging location within a lake (carbon signature, δ 13 C) and rank in the trophic chain (nitrogen signature, δ 15 N) (ref. 27 ). In both lakes, Benthics and Limnetics differed in δ 13 C (Apoyo: t (108)=4.65, P <0.0001; Xiloá: t (92)=3.67, P <0.0001; N =204) and differed in δ 15 N (Apoyo: t (108)=−3.79, P =0.0003; Xiloá: t (92)=−4.13, P <0.0001; N =204) ( Supplementary Fig. 3b,c ). Gut contents ( N =121) indicated that Limnetics consumed the lowest proportion of molluscs ( Supplementary Fig. 3h–m ). Overall, the relative variation between ecomorphs within lakes suggested that Limnetics occupied a higher trophic level (δ 15 N) and foraged in a different macrohabitat (δ 13 C) compared with Benthics. Population genetic differentiation The phenotypic divergence in morphology and ecology was accompanied by significant population genetic differentiation between the Limnetic ( A. zaliosus ) and each benthic species in Apoyo ( F ST =0.09–0.12, P <0.005; N =321) and significant population genetic differentiation among all species in Xiloá ( F ST =0.03–0.09, P <0.005; N =363) ( Supplementary Table 2 ). Therefore multiple lines of evidence—body shape, LPJ shape, weight and size, trophic level and diet, and population genetics—demonstrated a clear repeated independently evolved pattern of benthic–limnetic divergence within both crater lakes (fulfilling our criterion 1). Phenotypic parallelism To test whether this divergence is parallel across eco-morphological traits (criterion 2), we analyzed the vectors of phenotypic change [28] of combined eco-morphology: body elongation, LPJ weight, LPJ depth, LPJ width, LPJ length, δ 15 N and δ 13 C ( N =157). Path length between ecomorph centroids, or the amount of sympatric, multivariate phenotypic evolution, did not differ between the radiations across crater lakes (TrajSize=0.0860, P =0.896, permutation test). Similarly, the path direction through phenotypic space, which describes trait co-variation, did not differ between radiations (TrajDir=146.40, P =0.988, permutation test) ( Fig. 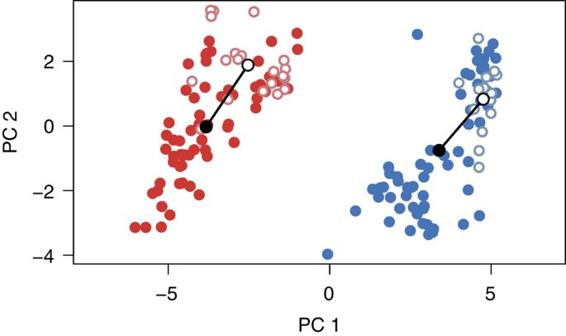Figure 3: Phenotypic trajectory analysis between Midas cichlid species flocks demonstrates parallel evolution. Each dot represents an individual after orthogonal projection of combined trophic and eco-morphological traits (body elongation index, LPJ weight, LPJ depth, LPJ width, LPJ length and stable isotope ratios of δ15N and δ13C) (N=157). The vectors of phenotypic difference between the centroids of Limnetic (open circle) and Benthic (black) phenotypic space did not differ in size or direction between the radiations of crater lakes Apoyo (red for Benthics, pink for Limnetics) and Xiloá (dark blue for Benthics, light blue for Limnetics). 3 ; see Supplementary Table 3 for each component separately). An analysis of diet across radiations also did not differ in amount (TrajSize=19.36, P =0.1350, permutation test) or direction (TrajDir=150.2, P =0.416, permutation test) of phenotypic evolution ( N =117; Supplementary Table 3 ). These elements strongly support parallel evolution along the benthic–limnetic axis in the two isolated crater lake radiations (fulfilling our criterion 2). Figure 3: Phenotypic trajectory analysis between Midas cichlid species flocks demonstrates parallel evolution. Each dot represents an individual after orthogonal projection of combined trophic and eco-morphological traits (body elongation index, LPJ weight, LPJ depth, LPJ width, LPJ length and stable isotope ratios of δ 15 N and δ 13 C) ( N =157). The vectors of phenotypic difference between the centroids of Limnetic (open circle) and Benthic (black) phenotypic space did not differ in size or direction between the radiations of crater lakes Apoyo (red for Benthics, pink for Limnetics) and Xiloá (dark blue for Benthics, light blue for Limnetics). Full size image Phylogenomics of speciation Multiple genomic analyses evidenced that this parallel evolution of radiations occurred independently across crater lakes (fulfilling our criterion 3). First, phylogenetic trees based on whole genome sequence of multiple individuals pooled per species ( =23.3 individuals per crater lake species, =47.5 individuals per Great Lake species) showed that the radiation in each crater lake was monophyletic (442,644 single nucleotide polymorphisms (SNPs) at 3 × minor allele coverage; maximum likelihood tree bootstrap proportion=100% for both crater lake, Fig. 4a ; maximum parsimony tree in Supplementary Fig. 5 ). The topology is robust to increasing the stringency of the minor allele coverage from 3 to 6 × ( Supplementary Fig. 4 ). In lake Apoyo speciation of the Limnetic A. zaliosus was the first divergence event relative to a monophyletic benthic flock. In contrast, in Xiloá the Limnetic ( A. sagittae ) was embedded in a paraphyletic benthic flock. Alternative topologies enforcing the Limnetic as the basal divergence in Xiloá were extremely unlikely (approximately unbiased test, P <2e−91; Supplementary Fig. 6 ). Perhaps because of the larger complement of species and genomic data in the current study, this differs from a previous genetic analysis that found A. sagittae to be the first divergence in Xiloá [29] . 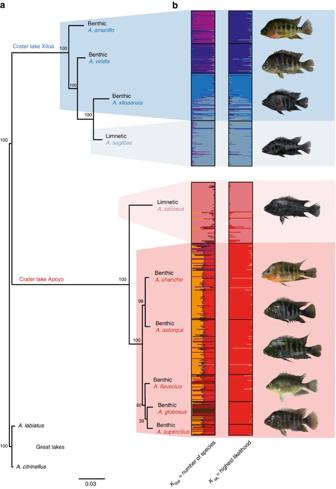Figure 4: Population genetic and phylogenetic analyses across two radiations. (a) A maximum likelihood phylogenetic tree based on a genome-wide matrix of 442,644 SNPs from pooled whole genome sequencing (N=327). There is strong evidence for a monophyletic origin (bootstrap proportions=100%) of the radiation in both crater lakes. (b) Population genetic analysis withouta prioriassignment to ecomorph and based on 14 microsatellite loci and two cluster analyses:KSppset to the number of species described within the lake (four in Xiloá, six in Apoyo), andKMLset to the highest likelihood, which reflects the best genetic clustering of data (three clusters in Xiloá, two clusters in Apoyo). Each horizontal bar represents an individual as its genotype is composed ofK-clusters (N=684). Figure 4: Population genetic and phylogenetic analyses across two radiations. ( a ) A maximum likelihood phylogenetic tree based on a genome-wide matrix of 442,644 SNPs from pooled whole genome sequencing ( N =327). There is strong evidence for a monophyletic origin (bootstrap proportions=100%) of the radiation in both crater lakes. ( b ) Population genetic analysis without a priori assignment to ecomorph and based on 14 microsatellite loci and two cluster analyses: K Spp set to the number of species described within the lake (four in Xiloá, six in Apoyo), and K ML set to the highest likelihood, which reflects the best genetic clustering of data (three clusters in Xiloá, two clusters in Apoyo). Each horizontal bar represents an individual as its genotype is composed of K -clusters ( N =684). Full size image Population genetics of speciation Individual-level analyses based on microsatellites confirmed the phylogenomic patterns: in Apoyo the best clustering ( K =2, N =321; Supplementary Table 4 ) separated the Limnetics ( A. zaliosus ) from all Benthics, while clustering based on number of species ( K =6) did not further distinguish benthic species; in Xiloá, the best supported clustering ( K =3, N =363) suggested considerable admixture between Limnetics ( A. sagittae ) and some Benthics (especially A. xiloaensis ) and clustering to the number of species ( K =4) did not further distinguish the Limnetics from Benthics ( Fig. 4b ). Therefore the extent and pattern of divergence order for Limnetics and Benthics differs between lakes. Our finding strongly suggests a non-parallel pattern of evolutionary divergence across the two radiations. Here we document a remarkable level of parallelism of ecological and morphological phenotype across two repeated radiations of crater lake cichlids. Unlike the grand scale parallel evolution in postglacial fishes [4] for which a role of secondary colonization was consistently important (for example, see refs 12 , 30 , 31 ), crater lake Midas cichlids have adaptively diversified independently and rapidly since colonization of Apoyo 10,000 years ago and Xiloá 5,400 years ago [16] , [21] , with no evidence for multiple colonizations. These results support a strong role of natural selection shaping similar ecomorphs in replicate because of similar environment and niche availability. This is a microevolutionary example of rewinding Gould’s tape [1] and resulting in the same outcome. Despite the strong parallelism in eco-morphology, we found striking non-parallelism in phylogenetic history and population genetic patterns across the two radiations. This agrees with previous research that did not identify parallel signals of genomic response to selection across these radiations [29] . It also may suggest a degree of predictability in divergence along the benthic–limnetic axis that might overcome particular lake-specific population-specific historical and demographic effects when a new and depauperate habitat is colonized. Our finding suggests that rapid parallel evolution of adaptive radiations can occur by non-parallel evolutionary routes. Specimen collection Midas cichlid fishes were collected from crater and great lakes by gill nets or by spearing in 2003, 2005, 2007 and 2010. Shortly after death, fish were digitally photographed in a standardized manner, on their right side with a scale bar. Muscle tissue and gut samples were collected and stored in pure ethanol. Fish heads or whole fish were taken as vouchers and stored in 70% ethanol. Species were initially taxonomically classified on site based on diagnostic keys and species descriptions [18] , [19] , [20] , [32] , [33] and later confirmed independently from photographs. Species were assigned to limnetic or benthic ecomorphs based on species descriptions and previous publications [16] , [18] , [19] , [20] , [34] and confirmed by a canonical variates analysis (see ‘Body shape and size’ under the methods section) that separated A. zaliosus in Apoyo and A. sagittae in Xiloá from all sympatric species (hereafter Limnetics= A. zaliosus and A. sagittae ; Benthics=all other species; Supplementary Fig. 1 ). All ten currently described species of the Midas cichlid species complex in lakes Apoyo and Xiloá were included in this study (see complete specimen list in Supplementary Data 1 ) plus 52 individuals of A. citrinellus and 43 A. labiatus from the Great Lakes Managua and Nicaragua for phylogenetic analysis (see Phylogenetic analysis under the methods section). The relevant authorities in the Nicaraguan Ministerio del Ambiente y Recursos Naturales approved all sampling. We compiled with the regulations of the Nicaraguan Ministerio del Ambiente y Recursos Naturales with regard to collections. Body shape and size Eighteen landmarks that describe body shape ( Fig. 2b ), plus two for size standard, were digitized in tpsDIG 2.12 (ref. 35 ) by a single investigator from the specimen photographs. Geometric morphometric analyses were performed in MorphoJ version 1.05c (ref. 36 ). A generalized least squares Procrustes superimposition [37] was conducted, in which the configuration of landmarks for each specimen was scaled to unit centroid size, translated to a common position and rotated to minimize distances between all landmark configurations. We applied a size correction to account for any allometric effects, that is, any dependence of body shape on absolute body size [38] , [39] . A multivariate regression of shape (Procrustes coordinates) on centroid size [40] was performed for each subgroup using a permutation test against the null hypothesis of independence (10,000 iterations). Size accounted for a significant proportion of the shape variation (2.21%, P <0.0001) so the regression residuals were then used for all subsequent geometric morphometric analyses. Principal components, canonical variates and discriminant function analyses were conducted to describe and visualize variation between individuals and groups, respectively, in morphological space. Shape differences were visualized with the thin plate spline technique. A univariate measure of fish body shape (Elongation Index [41] ) was calculated from body height (anterior insertion of dorsal fin to anterior insertion of pelvic fin) divided by standard length (top lip to intersection of caudal peduncle with the caudal fin), subtracted from 1 so that the index increases as body elongation increases (1−BH/SL). Linear measures were extracted from the digitized landmarks relative to size standard. LPJ shape and size LPJs were extracted from the fish heads, cleaned and dried, weighed on a microbalance, and measured for depth, width and length with digital callipers. Weight and size measures were corrected for body size (standard length) for all statistical analyses. T -tests between Benthic and Limnetic ecomorphs were conducted in JMP version 5.1 (ref. 42 ). For shape analyses, standardized photographs were taken from LPJs placed into an agarose gel such as the dentigerous area of the jaw was plane. Jaws were photographed from above with a perpendicular, fixed camera. Twenty-four landmarks (12 fixed and 12 semi-landmarks) that describe LPJ shape, including the dentigerous area ( Fig. 2d ) were digitized in tpsDIG version 2.12 (ref. 35 ) by a single investigator from the specimen photographs. Semi-landmarks were slid in tpsRelw version 1.49 (ref. 43 ) in orthogonal projection mode with 10 iterations. Semi-landmarks were then treated as true homologous landmarks in MorphoJ. Object symmetry was taken into account and the symmetric component of shape variation only was considered as our trait of interest [44] . A correction for allometric effects on LPJ shape was performed by regressing Procrustes coordinates on centroid size (3.22% explained; P <0.0001). Regression residuals were used in downstream analyses that were conducted analogous to the methodology for body shape. Diet and trophic analysis Stable isotope ratios of carbon (δ 13 C) and nitrogen (δ 15 N) were calculated from white muscle tissue (taken from severed heads, dorso-posterior near the lateral line) in the Limnological Institute, the University of Konstanz. All individuals included in diet and SIA analysis were adults that had been collected in a single sampling expedition (Nov.-Dec 2010). Samples were analyzed by gas chromatography combustion isotope ratio mass spectrometry (GC-C-IRMS). Values of δ 13 C were normalized for lipid content following [45] . T -tests between Benthic and Limnetic ecomorphs were conducted in JMP version 5.1 (ref. 42 ). Filled guts were dissected under a stereoscope by a single investigator. Gut contents were sorted into six categories: white algae, plant parts and seeds, Chara algae, insect pieces and larvae, mollusc shells, fish and fish parts. Volumes were visually estimated by comparing to a standard. Digested and unidentifiable food items were excluded. Schoener’s index [46] was calculated to obtain pair-wise species comparisons of diet overlap: C xy =1−0.5(∑| P xi – P yi |), where values range between 0 (no diet overlap) and 1 (complete diet overlap). Phenotypic change Parallelism of size and orientation of the difference in phenotype (body shape, elongation index, LPJ size and shape, stable isotopes) was analyzed using the phenotypic change vector analysis approach [28] , [47] implemented in R (ref. 48 ) using scripts provided by Adams and Collyer [28] . Analyses were conducted on both crater lake radiations simultaneously (factor 1=lake, factor 2=benthic or limnetic), with benthic species pooled. Briefly, we examined the evolutionary vectors in a principal component analysis by applying first a general linear model to calculate ecomorph centroids and then generating vectors between sympatric groups (following [28] , [49] , [50] ). This was done on all eco-morphological data pooled (resulting in seven PC dimensions) to obtain an integrative metric of multivariate evolutionary vectors and was also conducted on components of that data set separately (see Supplementary Table 3 ). The difference in magnitude and orientation of the vectors was compared statistically with the ‘residual randomization method’ [49] , [51] employing 999 permutations. Population genetics High-quality genomic DNA was extracted from fin tissue using the QiagenDNeasy Blood & Tissue Kit (Qiagen, Valencia, USA) following the manufacturer’s protocol. Samples were amplified and genotyped for 14 microsatellite loci: Abur28 (Forward: 5′-CGAAGCGCTTTAGTGGTTTC-3′, Reverse: 5′-CATCGCTCAGCTTTCTCCTC-3′), Abur45 (Forward: 5′-AGCAGTGGATGTGGCAGAG-3′, Reverse: 5′-TACAGGATGTGCCCCTCTC-3′), Abur82 (Forward: 5′-ACAAAGAGCATGCACAAATG-3′, Reverse: 5′-CAGGAGACACAGTGGGAGATG-3′), Abur151 (Forward: 5′-GTGAATGTGTGAGCGTGTCC-3′, Reverse: 5′-CAGATGCAAACAGCTCGAAG-3′) [52] , Unh002 (Forward: 5′-TTATCCCAACTTGCAACTCTATTT-3′, Reverse: 5′-TCCATTTCCTGATCTAACGACAAG-3′) [53] , Unh011 (Forward: 5′-GAAAGCCTT CCCAGAAGACC-3′, Reverse: 5′-CCTGACTGGCATTTGTAGCA-3′, Unh012 (Forward: 5′-GACCAGTCTTGGCTTCAGGA-3′, Reverse: 5′-CAGCATCAGCATCTCACACA-3′), Unh013 (ref. 54 ) (Forward: 5′-GCCACAGAAACAGACTTTAGCA-3′, Reverse: 5′-TGTCTTGGCATGCTTCTCAG-3′), M1M (=Acit1) (Forward: 5′-AAATGAGTTCAGCGATGGCTGAG-3′, Reverse: 5′-TGCACATCATGTCCGCCGAACA-3′), M2 (=Acit2) (Forward: 5′-GGCACTGAGGATTTATATTACAGG-3′, Reverse: 5′-GAGGTCCAGCTGAGAACAGGG-3′), M7 (=Acit3) (Forward: 5′-CTTAAGGTGTACCTGCTTAGC-3′, Reverse: 5′-GAGTGGGAAGACAGATGTTGAGG-3′), M12 (=Acit4) (ref. 55 ) (Forward: 5′-CCTTCCTACTAGTTAGTCTTTCAC-3′, Reverse: 5′-CACATAGCACAGTGCATTCACCC-3′), TmoM7 (Forward: 5′-CTGCAGCCTCGCTCACCACGTAT-3′, Reverse: 5′-CACCAGATAACTGCACAGCCCAG-3′) (ref. 56 ) and Burtkit F 474 (Forward: 5′-GATCTGGAGAATATGCACCTGGA-3′)/R672 (Reverse: 5′-ATCACTCTTGTGGATGGTTGGAG-3′) (ref. 57 ) using standard PCR conditions. For each locus, one primer was labelled with a NED, FAM or HEX fluorescent dye (Applied Biosystems) for subsequent visualization on an ABI 3130xl automatic capillary sequencer (Applied Biosystems). Fragment sizes were determined according to an internal GeneScan 500 ROX size standard (Applied Biosystems). Individual genotypes were scored with GeneMapper version 4.0 (Applied Biosystems). Electropherograms were controlled manually and low peaks (<20 relative fluorescent units) and ambiguous data were coded as missing. Individuals with missing data for more than five loci were excluded from further analysis. Data sets for all populations were checked for the effect of null alleles, erroneous stutter peaks and large allele dropout using Micro-Checker version 2.23 (ref. 58 ). For each population 1,000 randomizations were performed and the confidence interval was set to 95% to assess statistical significance. Genetic differentiation (Weir & Cockerham’s F -statistic) was calculated using the programme Microsatellite Analyzer (MSA) version 4.05 (ref. 59 ) and assessed with 10,000 genotype permutations. Structure version 2.3.3 (ref. 60 ) was used to estimate the most likely number of distinct population clusters as well as to assign individuals to these, with each lake analyzed separately. We assessed the likelihood of one to eight clusters without giving prior information of the species assignment of individuals, using an admixture model for correlated allele frequencies. This model seems biologically realistic due to the recent common ancestry of the crater lake populations [17] . For each K , five iterations were performed with a Markov chain Monte Carlo chain length of 500,000 steps following a burn-in period of 100,000 steps. The highest likelihood for the number of clusters was determined following [61] . Phylogenetic analysis High molecular weight DNA was pooled equimolar for multiple individuals (usually 26 individuals per species) for all species in crater lakes Xiloá, Apoyo and the great lakes ( Supplementary Table 5 ) to generate barcoded libraries following manufacturer’s protocols (Illumina Multiplexing Sample Preparation guide PE-930-1002). Libraries were pooled equimolar in sets of six or seven libraries for bridge amplification in cBOT (Illumina). Pooled libraries were sequenced in two runs across 13 flowcell lanes on an Illumina Genome Analyzer IIx (Genomics Centre, University of Konstanz). Paired-end sequencing of clustered template DNA was performed using four-color DNA Sequencing-By-Synthesis technology with 299 cycles (146 cycles for each end and 7 cycles for the barcode sequence). Sequencing quality was controlled with a PhiX lane. This generated 20,807,453–105,505,599 reads per species ( Supplementary Table 5 ). Shotgun genomic data are deposited in the European Nucleotide Archive. The raw reads of each species were first trimmed to remove the adaptors and the low quality bases using CLC Genomics Workbench version 5.5.1 and then mapped to the A. citrinellus genome (shotgun and assembled data are deposited in the European Nucleotide Archive), using Bowtie2 version 2.0.6 with paired-end mode [62] . The raw mapping results were converted to BAM format using Samtools version 0.1.18 (ref. 63 ) in which (1) the mapped reads were sorted by their positions in the genome, (2) mapping quality was required to be at least 20 to exclude low quality/ambiguous mapped reads. To identify SNPs among species, a mpileup format file ( http://samtools.sourceforge.net/samtools.shtml ), which includes mapping information across all the species, was generated using Samtools. An in-house Perl script was written to extract the intra- and inter-species SNP information. Specifically, we first extracted the intraspecific SNPs by requiring (1) the coverage of the sites to be >10 times, if not the site was coded as missing data ‘N’, (2) the minimum coverage of the minor allele of in a SNP site was required to be at least 3 × , which if present resulted in a standard IUPAC nucleotide code. We required that a SNP site should be shared by at least eight species to minimize the impact of missing data [64] . Using these criteria, a matrix was generated of 442,644 SNPs across 12 species. Alternative matrices were also analyzed with increased alternative allele coverage of ≥6 × . We constructed a phylogeny using RaxML (ref. 65 ) with General Time Reversible and Gamma model of nucleotide evolution model [66] . The robustness of the phylogeny was evaluated by 100 ‘rapid-bootstrap’ replicates [65] . The maximum likelihood topology was compared with four alternative topologies in CONSEL version 0.20 (ref. 67 ). A maximum parsimony analysis of the SNP matrix was conducted in PAUP* version 4.0b10 (ref. 68 ) using heuristic searches with 10 random-addition-sequence replicates and the tree bisection-reconnection branch swapping option. Bootstrap support values were calculated with 2,000 replicates. Accession codes: The short read DNA sequences for population genomics have been deposited in the European Nucleotide Archive (ENA) under the accession code PRJEB6990 . The A. citrinellus draft genome version 5 (assembly and short reads) has been deposited in the European Nucleotide Archive (ENA) under the accession code PRJEB6974 . How to cite this article: Elmer, K. R. et al. Parallel evolution of Nicaraguan crater lake cichlid fishes via non-parallel routes. Nat. Commun. 5:5168 doi: 10.1038/ncomms6168 (2014).